Proteome-wide selected reaction monitoring assays for the human pathogenStreptococcus pyogenes Selected reaction monitoring mass spectrometry (SRM-MS) is a targeted proteomics technology used to identify and quantify proteins with high sensitivity, specificity and high reproducibility. Execution of SRM-MS relies on protein-specific SRM assays, a set of experimental parameters that requires considerable effort to develop. Here we present a proteome-wide SRM assay repository for the gram-positive human pathogen group A Streptococcus. Using a multi-layered approach we generated SRM assays for 10,412 distinct group A Streptococcus peptides followed by extensive testing of the selected reaction monitoring assays in >200 different group A Streptococcus protein pools. Based on the number of SRM assay observations we created a rule-based selected reaction monitoring assay-scoring model to select the most suitable assays per protein for a given cellular compartment and bacterial state. The resource described here represents an important tool for deciphering the group A Streptococcus proteome using selected reaction monitoring and we anticipate that concepts described here can be extended to other pathogens. Bacterial infections are a major cause of disease and mortality aggravated by the emerging resistance to antibiotics. During an infection, pathogenic bacteria can rapidly alter their proteome composition to adapt to hostile environments and evade immune response [1] , [2] , [3] , [4] . How the bacteria regulate their proteome composition in vivo to accomplish host environment adaption and immune response evasion is, however, still unclear. Quantitative and comprehensive in vivo proteome-wide analysis of large cohorts of clinically isolated bacterial strains would considerably improve our understanding of how these processes are accomplished and how they are influenced by underlying genetic differences and environmental factors. For example, advances in understanding underlying genetic differences between clinical group A Streptococcus (GAS) strains have revealed that mutations in the regulatory system covRS is linked to a severe disease outcome and as reviewed by Cole et al. [5] Modern proteomics technologies allow quantitative measurement of the vast majority of proteins in bacterial proteomes [6] . The conceptual advance of directed mass spectrometry (MS) technologies using liquid chromatography coupled to tandem MS (LC–MS/MS) [7] has resulted in several proteome-wide absolute quantification studies of how bacteria adapt to new environments in vitro [8] , [9] , [10] . The development of selected reaction monitoring (SRM)-MS analysis has recently become a viable complement to data dependent and directed MS analysis because data sets with unprecedented reproducibility across multiple samples and a large dynamic range can be achieved. SRM is a targeted MS technology where preselected pairs of peptide precursor ion and fragment ion mass masses, also known as transitions, are explicitly monitored over time in a triple quadrupole (QQQ) MS instrument. The non-scanning mode of measurement of the most intense peptides and peptide fragments for each protein results in the lowest limit of detection of any LC-based MS technique. Using SRM to study pathogen virulence mechanisms is attractive as bacterial proteomes have an estimated dynamic range of 4–5 orders of magnitude [10] , which is smaller than the linear dynamic range of SRM [11] A key characteristic of SRM-MS analysis is the accurate protein quantification capability, where the quantification variance is similar to enzyme-linked immunosorbent assay in bacterial proteomes [12] . The accurate protein quantification capability along with the reproducible mode of analysis results in comprehensive data matrices (protein quantity versus sample) with very few missing values, as the same peptide species are measured in all samples [13] , [14] . The consistency and completeness of such data sets is important for the analysis of, for example, large collections of clinically isolated strains or for studying small genetic differences resulting in single-amino acid substitutions. The execution of SRM experiments is dependent on a priori knowledge regarding which peptides and transitions to target. This knowledge is typically obtained by creating deep proteome maps using multidimensional peptide fractionation strategies followed by data-dependent LC–MS/MS analysis. From such proteome maps, proteotypic peptides (PTP’s) uniquely identifying proteins of interest, and suitable transitions are selected and optimized [15] . The transitions are subsequently used by QQQ mass spectrometers, where peptide ions are isolated in the first quadrupole, fragmented in the second and the resulting peptide fragments are isolated and monitored in the third quadrupole, providing a high-degree of selectivity and sensitivity for the detection of the targeted peptides. Several transitions per peptide are commonly used to increase the confidence level that the targeted peptide is in fact identified and accurately quantified. Sets of transitions for a single precursor peptide along with the precise retention time (RT) are collectively referred to as an SRM assay. The limited availability of SRM assays is a prohibitive bottleneck for carrying out SRM-MS analyses and necessitates time consuming and expensive SRM assay development. Although there is currently a considerable amount of effort put into the construction of large-scale transitions atlases to facilitate the step from selecting target proteins to actually measuring them [16] , a proteome-wide repository for a bacterial pathogen has not been reported to date. In the work described here we demonstrate the construction of a proteome-wide SRM assay repository for the important human pathogen GAS. GAS is a gram-positive bacterium responsible for common and relatively mild clinical conditions such as pharyngitis and streptococcal skin infections [17] , [18] . GAS can also cause severe and potentially life-threatening conditions such as septic shock and necrotizing fasciitis, resulting in >500,000 deaths every year, thus making GAS one of the more important human pathogens. The work described here outlines a multi-layered approach to generate SRM assays for 10,412 distinct GAS peptides. To improve the usability of the repository we performed extensive testing of all SRM assays in different bacterial states and cellular compartments. Based on the performance of the individual assays as a function of biological matrix, we calculated an assay score based on a rule-based assay-scoring model. This score ranks individual assays based on their detectability. The assay score ranked, proteome-wide SRM assay repository presented here provides an important resource for understanding GAS proteome spatial distribution, organization of related protein functions and protein abundance range. Furthermore, we define a transportability index indicating the portability of individual SRM assays across related genomes. We anticipate that the data described here will become an important resource for understanding GAS biology and that they can be used as a basis for the construction of SRM-wide assay repositories for other pathogens, emerging pathogens and commensal bacteria. Constructing a proteome-wide GAS SF370 SRM assay repository We selected GAS SF370 as the model strain for the construction of a proteome-wide GAS SRM assay repository. Previous LC–MS/MS analysis on GAS SF370 resulted in the identification of 946 of the 1,905 GAS SF370 open reading frames (ORFs) [7] . The data resulting from these measurements were stored in a publically available instance of PeptideAtlas [19] . In this study we expanded the available PeptideAtlas instance by resorting to sub-cellular fractionation from several GAS strains grown under various environmental conditions ( Fig. 1a ). In total, 433 high-resolution LC–MS/MS measurements using 231 unique protein pools resulted in the identification of 8,320 PTP’s for GAS. The PTP’s were ranked according to decreasing extracted ion chromatogram (XIC) intensities, estimating protein abundance as previously described [10] , and served as the basis for the construction of the proteome-wide SRM assay repository. 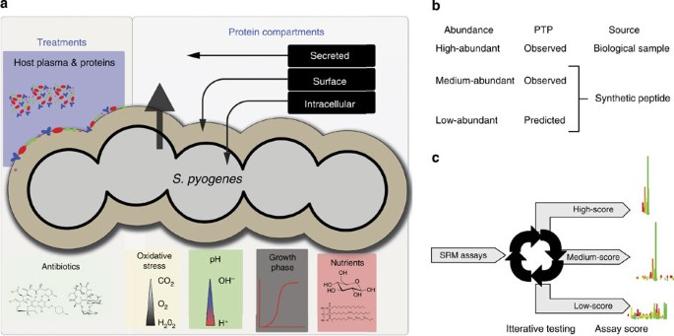Figure 1: Construction of a proteome-wide SRM assay repository. (a) Graphical representation of the enriched Group A Streptococci (GAS) cellular compartments. Repeated enrichment of protein pools from the cellular compartments and bacterial states were digested using trypsin and analysed by LC tandem MS (LC–MS/MS). (b) Outline of the strategy used to construct a spectral library from where the low-scoring SRM assays were extracted. For high-abundant PTP’s the SRM assays were determined directly in biological samples, whereas for medium- and low-abundant PTP peptides were synthesized and analysed with LC–MS/MS. (c) To increase the confidence of the individual SRM assays the low-scoring SRM assays were tested extensively in complex mixture of GAS tryptic digest using SRM. Figure 1: Construction of a proteome-wide SRM assay repository. ( a ) Graphical representation of the enriched Group A Streptococci (GAS) cellular compartments. Repeated enrichment of protein pools from the cellular compartments and bacterial states were digested using trypsin and analysed by LC tandem MS (LC–MS/MS). ( b ) Outline of the strategy used to construct a spectral library from where the low-scoring SRM assays were extracted. For high-abundant PTP’s the SRM assays were determined directly in biological samples, whereas for medium- and low-abundant PTP peptides were synthesized and analysed with LC–MS/MS. ( c ) To increase the confidence of the individual SRM assays the low-scoring SRM assays were tested extensively in complex mixture of GAS tryptic digest using SRM. Full size image The construction of the proteome-wide SRM assay repository relied on a two-legged strategy. The first leg, outlined in Fig. 1b , involved the construction of SRM assays based on a MS/MS spectral library. We constructed the spectral library for high abundant PTP’s identified by several MS/MS spectra from the large-scale proteome inventory as previously described [20] . For PTP’s without a sufficient number of fragment ion spectra to create a reliable spectral library, the corresponding PTP’s were chemically synthesized. For proteins that remained undetected in the proteome mapping data sets we predicted the most suitable PTP’s using APEX [21] and synthesized corresponding peptides, generating in total 2,489 synthetic peptides. The synthesized peptides were analysed by shotgun MS/MS and the resulting data were amended to the spectral library. The strongest conserved transitions and the RT were extracted from the spectral library and stored, enabling RT normalized SRM assays to be downloaded directly into the SRM methods used by the MS [22] . The efforts resulted in 10,412 SRM assays and the transitions were ranked according to intensity as described earlier [20] . The second leg included iterative testing of the assays with SRM using a QQQ instrument to increase the confidence of individual SRM assays ( Fig. 1c ). We tested 7,621 distinct peptide sequences with their corresponding SRM assays, represented by a total of 79,277 transitions, in cell lysates from GAS grown under different conditions. The conditions included different growth phases, oxidative stress, exposure to human plasma supplement or antibiotics ( Fig. 1a ). All SRM assays were tested at least two times and several more than hundred times ( Fig. 2a ), resulting in 957,850 individual ion chromatograms. The most frequently observed SRM assays and the most intense transitions associated with them were ranked as described previously [20] . We used this information to build an SRM assay score using a rule-based scoring model. The model divides the assays into three categories, low-, medium- and high-scoring. The scoring indicates the ability of an SRM assay to detect the corresponding peptide in tryptic GAS digests from cellular compartments and different bacterial states ( Fig. 1c ). The major assay score parameter is based on the SRM false discovery rate (FDR) thresholds of peptide identification in complex biological peptide mixtures. The high-scoring assays represent cases where the peptide was detected with high confidence in complex GAS peptide mixtures (FDR of ≤1%). The medium-scoring assays represent cases where the peptide was detected with lower confidence (FDR 1>2%). These SRM assay score categories received and arbitrary score of 100 and 50, respectively. SRM assays developed on synthetic peptides were included in the medium-scoring SRM assays. The fine-tuning of the assay score within these two categories was based on the number of times the peptides were observed, minus the number of attempted observations divided by two. Thus, the higher the frequency with which an SRM assay was observed with high probability, the higher the assay score. The low-scoring SRM assays represent cases where the peptide remained undetected in complex GAS peptide mixtures. These SRM assays were scored based on the number of transitions per SRM assay, which positively influences the low-scoring SRM assay scores to a moderate extent. Hence, peptides represented by low-scoring SRM assays were never observed in streptococcal protein extracts. High- and medium-scoring assays were measured in good agreement with the synthetic SRM assays, but with different FDR thresholds. 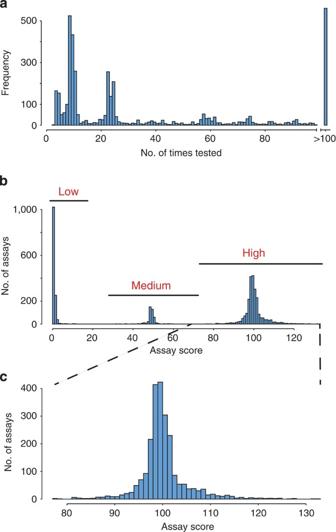Figure 2: Rule-based assay score modelling can select high performing assays depending on cellular compartment and cellular state. SRM assays were tested repeatedly in mixtures of GAS tryptic digests from different sub-cellular compartments and bacterial states. (a) Statistics over the repetitive testing of all SRM assays. They-axis shows the frequency of the number of times a SRM assay was tested. (b) The assays were divided up into three categories, low-, medium- and high-scoring SRM assays based on a rule-based assay score model. In summary, the higher the frequency with which an SRM assay was observed with high probability, the higher the assay score. (c) Assay score distribution for high-scoring SRM assays. Figure 2b shows the current distribution of GAS SRM assays in the three categories, demonstrating that we can preferentially select suitable assays per protein using the rule-based assay-scoring model. As the number of observations increases over time, we anticipate continued improvement of the assay score prediction. In total we have defined 2,731 SRM assays with a medium- or high-score, targeting 1,332 proteins. Out of these 1,201 (63.0% of total ORF’s) were detected in complex mixtures (high-scoring SRM assays). Twenty-three percent of the predicted ORF’s were associated with low-scoring SRM assays. For the majority of applications, the complete set of SRM assays provided in this study are typically not included for analysis. The developed assays score provides means to select the suitable SRM assays depending on targeted proteins and type of experiment and represent a useful strategy for prioritizing among the SRM assays. Figure 2: Rule-based assay score modelling can select high performing assays depending on cellular compartment and cellular state. SRM assays were tested repeatedly in mixtures of GAS tryptic digests from different sub-cellular compartments and bacterial states. ( a ) Statistics over the repetitive testing of all SRM assays. The y -axis shows the frequency of the number of times a SRM assay was tested. ( b ) The assays were divided up into three categories, low-, medium- and high-scoring SRM assays based on a rule-based assay score model. In summary, the higher the frequency with which an SRM assay was observed with high probability, the higher the assay score. ( c ) Assay score distribution for high-scoring SRM assays. Full size image SRM assay score biases As the dynamic range of SRM is higher than the estimated dynamic range for microbial proteomes, we anticipate that the undetected proteins are not related to limitations in sensitivity of the method or the dynamic range of the sample. To estimate method biases between detected and undetected proteins we compared enrichment of the proteins associated with the different assay score categories to a number of parameters such as protein length, protein conservation and functional classification. Apart from the three major tendencies between the scoring categories we discovered surprisingly few biases. Firstly, we compared the relationship between proteins associated with high SRM assay scores and protein abundance estimated from extracted XIC from the shotgun proteome inventory established in the beginning of the study. XIC of the identified proteins with 1% FDR were extracted and summed up and associated to the SRM assay score categories ( Fig. 3a ). On average 91.6% of the identified XIC were associated with proteins with at least one high- or medium-scoring SRM assay. 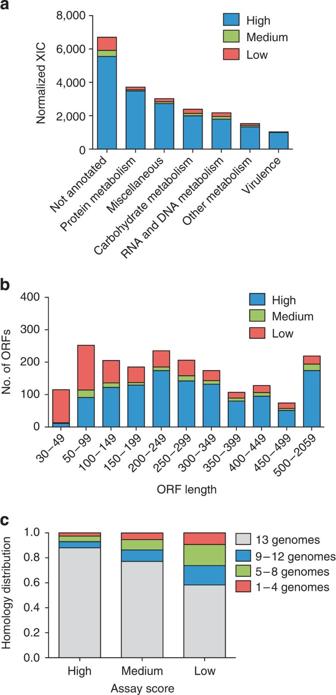Figure 3: Protein identification biases across functional categories and ORF properties. Iterative testing of the developed SRM assays in complex biological mixtures of GAS tryptic digests resulted in subdivision of the proteins into three SRM assays-score categories; proteins with low-, medium- or high-scoring SRM assays. Using the SRM assay score categories we determined biases among associated proteins within the three categories. (a) Proportion of XIC intensities associated with proteins with at least one high or medium-scoring SRM assay or proteins with low-scoring SRM assays. NMPDR was used to categorize proteins; protein metabolism includes categories amino acids and derivatives and protein metabolism; miscellaneous includes categories clustering-based sub-systems, miscellaneous, phages, prophages, transposable elements, plasmids, regulation and cell signalling, respiration, stress response, cell division and cell cycle and cell wall and capsule; carbohydrate metabolism includes category carbohydrates; RNA and DNA metabolism includes categories nucleosides and nucleotides, DNA metabolism and RNA metabolism; other metabolism includes categories phosphorus metabolism, potassium metabolism, fatty acids, lipids and isoprenoids, cofactors, vitamins, prosthetic groups and pigments, sulphur metabolism, iron acquisition and metabolism, nitrogen metabolism, membrane transport and metabolism of aromatic compounds virulence includes categories virulence and virulence, disease and defence. (b) Genome-wide correlation between SRM assay score and ORF length. (c) Correlation between SRM assay score and relative degree of protein conservation across 13 GAS strains as determined with TOP-BLAST hits with SF370 as reference. Figure 3a does not include the proteins that were exclusively identified using SRM. The overlap between proteins with high assays score and proportion of XIC indicates that SRM can recapture the vast majority of identified proteins from the large shotgun proteome inventory analysis and in addition identify additional proteins. In the SRM experiments, however, no additional offline peptide separation was performed, as was the case when the shotgun proteome inventory was constructed. Figure 3: Protein identification biases across functional categories and ORF properties. Iterative testing of the developed SRM assays in complex biological mixtures of GAS tryptic digests resulted in subdivision of the proteins into three SRM assays-score categories; proteins with low-, medium- or high-scoring SRM assays. Using the SRM assay score categories we determined biases among associated proteins within the three categories. ( a ) Proportion of XIC intensities associated with proteins with at least one high or medium-scoring SRM assay or proteins with low-scoring SRM assays. NMPDR was used to categorize proteins; protein metabolism includes categories amino acids and derivatives and protein metabolism; miscellaneous includes categories clustering-based sub-systems, miscellaneous, phages, prophages, transposable elements, plasmids, regulation and cell signalling, respiration, stress response, cell division and cell cycle and cell wall and capsule; carbohydrate metabolism includes category carbohydrates; RNA and DNA metabolism includes categories nucleosides and nucleotides, DNA metabolism and RNA metabolism; other metabolism includes categories phosphorus metabolism, potassium metabolism, fatty acids, lipids and isoprenoids, cofactors, vitamins, prosthetic groups and pigments, sulphur metabolism, iron acquisition and metabolism, nitrogen metabolism, membrane transport and metabolism of aromatic compounds virulence includes categories virulence and virulence, disease and defence. ( b ) Genome-wide correlation between SRM assay score and ORF length. ( c ) Correlation between SRM assay score and relative degree of protein conservation across 13 GAS strains as determined with TOP-BLAST hits with SF370 as reference. Full size image The second tendency relates to protein length where we observed that proteins with low-scoring SRM assays were predominately short compared with proteins with medium- and high-scoring SRM assays ( Fig. 3b ). In contrast, proteins with high-scoring SRM assays were predominately long, indicating, as expected, that a larger number of PTP’s to choose from per protein is beneficial for SRM analysis ( Fig. 3b ). The third tendency relates to protein conservation among the GAS genomes where relatively many proteins with low-scoring SRM assays are less conserved or unique compared with other GAS strains ( Fig. 3c ). Around 58% of the protein sequences associated with low-scoring SRM assays are conserved across all 13 genomes tested ( Supplementary Table S1 ). In contrast, 88% of the high-scoring SRM assays were associated to conserved proteins conserved across all 13 genomes, indicating that conserved proteins are expressed at higher frequency than non-conserved protein sequences under the tested conditions ( Fig. 3c ). Collectively, we note that the extensive MS analysis of GAS described here using two different MS platforms provide a large degree of overlap. Proteins with low-scoring assays tend to be less suitable for MS analysis by any method, as they were short and thus contain fewer suitable PTP’s. In addition, we observe an overrepresentation of proteins with high-scoring assays among conserved protein sequences within the GAS protein universe. It is likely that the protein sequences with exclusively low-scoring SRM assays are not expressed under the tested growth conditions. Membrane proteins were not specifically addressed in the sub-cellular fractionation, however, we observe no overall bias against membrane proteins. Nevertheless, detection of certain membrane protein species may require specific digestion/extraction methods [23] , [24] . Spatial distribution of proteins with high-scoring assays The iterative testing of the developed SRM assays on more than 540 LC–SRM-MS measurements represents a comprehensive proteome-wide targeted measurement of the GAS SF370 encoding genome. As we tested the SRM assays in enriched fractions of the intracellular, surface-associated and secreted protein pools we could also estimate the predominant localization for proteins associated with high-scoring SRM assays ( Fig. 4 ). The majority of the proteins, 934 proteins were predominately present in the intracellular pool ( Fig. 4a ). A smaller fraction, 115 and 28 proteins, were predominately found in the surface-associated and secreted protein pools, respectively ( Fig. 4c ) leaving 124 proteins that were relatively evenly split between two or more compartments ( Fig. 4e ). 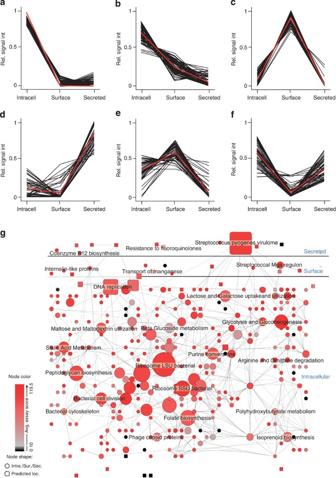Figure 4: Spatial distribution of proteins with high-scoring SRM assays. Testing of all SRM assays in three sub-cellular compartments enabled the construction of a sub-cellular distribution map for the proteins with high-scoring assays. By usingk-mean clustering, the expression profiles were split into six different clusters: (a,b) predominately intracellular proteins, (c) surface-associated proteins, (d) secreted proteins and (e,f) proteins with split sub-cellular compartmentalization. Black lines ina–frepresent the relative protein compartment signal and the red lines represent the average distribution of the clusters. Subsequently the identified proteins were grouped into NMPDR sub-systems and visualized using Cytoscape. (g) Outline of the GAS proteome network topology, where circles represent NMPDR sub-systems where all proteins predominantly have the same sub-cellular location, secreted, surface-associated or intracellular, according to the sub-cellular protein profiles in (a,d). Rectangles represent NMPDR sub-systems where an equal number of members have opposing sub-cellular location profiles. The localization of the rectangles in the network is influenced by the edges, which represent protein members that belong to more than one NMPDR sub-system. Increasing node size represents increasing number of member proteins. The colour represents average SRM assay score, where red indicates NMPDR sub-systems with high-average SRM assay score and black indicating NMPDR sub-systems with low average SRM assays score. For full details of NMPDR sub-systems seeSupplementary Fig. S1. Figure 4: Spatial distribution of proteins with high-scoring SRM assays. Testing of all SRM assays in three sub-cellular compartments enabled the construction of a sub-cellular distribution map for the proteins with high-scoring assays. By using k -mean clustering, the expression profiles were split into six different clusters: ( a , b ) predominately intracellular proteins, ( c ) surface-associated proteins, ( d ) secreted proteins and ( e , f ) proteins with split sub-cellular compartmentalization. Black lines in a – f represent the relative protein compartment signal and the red lines represent the average distribution of the clusters. Subsequently the identified proteins were grouped into NMPDR sub-systems and visualized using Cytoscape. ( g ) Outline of the GAS proteome network topology, where circles represent NMPDR sub-systems where all proteins predominantly have the same sub-cellular location, secreted, surface-associated or intracellular, according to the sub-cellular protein profiles in ( a , d ). Rectangles represent NMPDR sub-systems where an equal number of members have opposing sub-cellular location profiles. The localization of the rectangles in the network is influenced by the edges, which represent protein members that belong to more than one NMPDR sub-system. Increasing node size represents increasing number of member proteins. The colour represents average SRM assay score, where red indicates NMPDR sub-systems with high-average SRM assay score and black indicating NMPDR sub-systems with low average SRM assays score. For full details of NMPDR sub-systems see Supplementary Fig. S1 . Full size image To visualize the proteome distribution we used Cystoscape [25] with the Cerebral [26] plugin ( Fig. 4g , Supplementary Fig. S1 ). The proteins were grouped according to cellular functions using the National pathogen microbe data resource (NMPDR) sub-system information [27] (now part of PATRICs Bioinformatics Resource Center [28] ) and selected cellular location for the individual functional categories based on the protein expression profiles shown in Fig. 4a–d , represented as circles in Fig. 4g . Cellular functional categories containing either proteins with contradicting cellular location from cluster Fig. 4e or different proteins with contradicting cellular location were considered to have unknown localization and are represented as rectangles in Fig. 4g . The size of the circles/rectangles indicates the number of member proteins ranging from 1 to 34. The edges between the circles/rectangles represent protein members that belong to more than one NMPDR sub-system, whereas the location of the rectangles within the network view is influenced by the edges. The colour scheme represents continuous decreasing average SRM assay score, where red indicates NMPDR sub-systems with high-average SRM assay score (>119) and black indicating proteins with predominately low-scoring SRM assays (<10). It can be noted that the majority of circles and rectangles are red, demonstrating the coverage of high-scoring assays across the GAS proteome. Several black protein groups were not detectable under the tested growth conditions. In general these sub-systems contain relatively few members. In summary, the iterative testing of the SRM assays in three sub-cellular compartments provides an overview of the sub-cellular protein distribution for GAS strain SF370. The majority of the nodes have a relatively high proportion of high-scoring SRM assays. More information regarding the sub-cellular localization for individual proteins can be found in Supplementary Data 1 . Transportability of SRM assays across the GAS pan-genome and related species We used GAS SF370 as a model strain when developing the proteome-wide SRM assay repository. However, as there is substantial genetic variation within and between genomes from different GAS serotypes [29] , [30] , [31] , [32] , it is important to know which SRM assays target proteins in other GAS strains. To explore the transportability of this resource to other GAS strains and closely or distantly related species, we selected in total 75 taxa of low-GC Gram-positive bacteria, Firmictutes, ( Supplementary Fig. S2 ) and mapped medium- and high-scoring SF370 assays onto respective genome. To estimate the taxon evolutionary relationship, a phylogenetic tree was constructed based on respective rpoB gene sequence ( Supplementary Fig. S2 ). There was a large attrition of assays with increasing evolutionary distance ( Fig. 5a ) and depending taxonomic rank ( Fig. 5b ). Nevertheless, transportability within the species rank was high ( Fig. 5b ) with average genome coverage’s of 59–70% (1,167–1,332 ORFs) demonstrating that the developed SRM assays will target a majority of the currently defined GAS pan-genome products independent on serotype or strain ( Fig. 5c ). Transportability in the genus rank was the most diverse (8–31% genome coverage) ( Fig. 5b ) with Group C streptococci genomes having the highest degree of average coverage and also being the closest related taxa based on rpoB homologies ( Fig. 5a ). 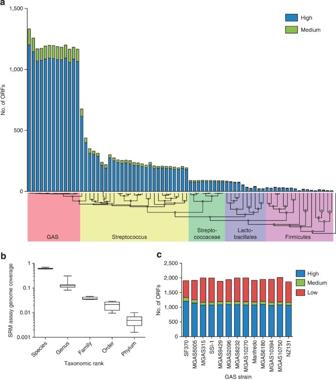Figure 5: SRM assay transportability to related species. All SRM assays were developed on basis of the GAS strain SF370 genome. The degree of SRM assay transportability within selected species was determined phylogeny clustering of respectiverpoBgene and mapping medium- and high-scoring SRM assays on to respective genome. (a) Transportability for the SRM assays across 75 genomes within the Firmicutes phylum. (b) Average ORF genome coverage of high- and medium-scoring SRM assays within taxonomic ranks. Boxes extend from the 25thto 75thpercentiles and error bars represent minimum to maximum values. (c) View of SRM assay transportability for 13 GAS genomes deposited in the public domain. Figure 5: SRM assay transportability to related species. All SRM assays were developed on basis of the GAS strain SF370 genome. The degree of SRM assay transportability within selected species was determined phylogeny clustering of respective rpoB gene and mapping medium- and high-scoring SRM assays on to respective genome. ( a ) Transportability for the SRM assays across 75 genomes within the Firmicutes phylum. ( b ) Average ORF genome coverage of high- and medium-scoring SRM assays within taxonomic ranks. Boxes extend from the 25 th to 75 th percentiles and error bars represent minimum to maximum values. ( c ) View of SRM assay transportability for 13 GAS genomes deposited in the public domain. Full size image To address the identity of proteins with transferable assays we calculated the number of species with at least a single high-scoring peptide belonging NMPDR sub-system. We note that the most frequent NMPDR functions with SRM assays with high-degree of transportability are as expected ribosomal proteins, universal GTPases and proteins involved in central metabolism. In contrast, the NMPDR sub-sytems with lowest level of transportability are Phage capsid proteins, Custered, Regularly Interspaced Short Palindromic Repeats (CRISPR) associated proteins and S. pyogenes Virulome (see Supplementary Fig. S3a,b for more information). The SRM assay transportability is an important parameter when targeting GAS proteins in microbial communities as for example in the oral cavity where many bacterial species are present [33] . SRM assay repository and availability The availability of the SRM assays (transitions, RT and collision energy), their NMPDR sub-systems, measured sub-cellular localization and degree of transferability is found in Supplementary Data 2 . The full list of SRM assays can be downloaded from the PeptideAtlas Public SRM Transition Lists at https://db.systemsbiology.net/sbeams/cgi/PeptideAtlas/GetTransitionLists under the accession number PATR00014. SRM is a targeted proteomics technology capable of accurate and reproducible quantification of proteins in complex samples. SRM has a dynamic range that is consistent with the analysis of microbial proteomes. In this paper, we provide a comprehensive proteome-wide SRM assay repository resource for the important human pathogen GAS, to remove a considerable bottleneck in the SRM workflow. We used a new proof-of-concept assays score to rank assays associated to a particular protein, based on the ability to detect assays in the tested conditions, resulting in 2,731 medium- or high-scoring assays covering 1,332 of 1,905 ORFs in the reference strain SF370. Any laboratory with access to QQQ mass spectrometers can use the SRM assays described in this manuscript to in a multiplexed manner quantify GAS proteins of interest. The additional use of stable isotope labelled reference peptides enables absolute protein copy number per cell estimations as previously described [10] . Searching for biases between proteins with low-, medium- and high-scoring SRM assays reveal that the majority of proteins with exclusively low-scoring assays tend to be shorter, less well annotated and less conserved among GAS strains. In contrast, the proteins associated with high-scoring SRM assays are longer, well annotated and conserved. As the dynamic range of SRM is higher than the dynamic range of the sample protein abundance we estimate that the missing proteins are due to lack of expression or proteins lost in the protein enrichment, digest or MS analysis. In addition, as the elution profile for tryptic peptides is not evenly distributed across the LC–chromatograms, certain peptides in particularly crowded areas are harder to confidently identify because of the presence of interfering signals from other high abundant peptides [20] . Although the outlined work resulted in considerable coverage over the GAS SF370 genome, still a considerable proportion of predicted GAS genes remained elusive. The iterative testing of >7,500 distinct peptide sequences with corresponding SRM assays provides an indication of the spatial distribution of the GAS proteome. This exemplified by high enrichments of cell walled anchored proteins in the surface compartment, and virulence factors in the secreted fraction. However, a substantial number of ribosomal proteins and central metabolic enzymes are detected in the extracellular fractions. In fact, around 10% of the detected proteins displayed similar abundance levels in >1 cellular compartment. There are probably several reasons for this, which are difficult to distinguish. Similar phenomena has been described earlier [34] , [35] , [36] , and could be explained by spontaneous cell lysis or artifacts related to experimental procedures. However, it is also likely that certain proteins are present in >1 cellular compartment natively. This has been described in detail for several GAS proteins as examples, glycolytic proteins implicated as virulence factors located on the surface [37] , [38] , [39] or cell wall anchored proteins proteolytically released into the growth media [40] , [41] , [42] . We believe the SRM assay repository will become a useful resource for addressing central medical and molecular microbiological related questions regarding GAS in general as the transportability of the SRM assays across the known GAS protein universe was high. Relatively little effort is required to also cover other strain-specific SRM assays in the respiratory. Defining GAS proteome composition differences between clinical isolates and mutant strains in vitro and in vivo are examples of how SRM assay repository could be used. Awareness of SRM assay transportability to closely related species is essential if targeting GAS proteins in microbial ecologies, such as in pharyngitis in vivo . In conclusion, we have in this work provided a proteome-wide SRM assay repository resource for one of the most important human pathogens to facilitate SRM-MS analysis for this bacterium. As several assays can be transported to other species we expect that the reach of the resource extend beyond GAS. We believe that the iterative testing of all SRM assays and the construction of a novel SRM assay score model along with estimating protein-specific biases for the differential scoring SRM assays increases the usefulness of the described resource. Bacterial culture conditions S. pyogenes M1 strains SF370, MGAS5005 and AP1 (strain 40/58 from the WHO Collaborating Centre for Reference and Research on Streptococci, Prague, Czech Republic) was cultured (37 °C; 5% CO 2 ) in C-medium [43] , Todd-Hewitt (TH) broth (Difco Laboratories) or in TH with supplements as indicated below or in Protein-reduced TH broth [36] for secreted protein isolation. Supplements were added to TH as indicated at the following concentrations: 1, 5, 10, 20 or 50% (V/V) citrate-treated human plasma (Skåne University Hospital, SUS) 50% (V/V) citrate-treated mouse plasma from CD1 mice (SeraLab), 4 mg ml −1 human serum albumin (Sigma-Aldrich), 4 mg ml −1 essentially fatty acid free (~0.005%) human serum albumin (Sigma-Aldrich), 0.3 mg ml −1 human fibrinogen (Sigma-Aldrich), 1.2 mg ml −1 human IgG (Sigma-Aldrich), rifampicin at the following concentrations 0.25, 1.25, 2.5, 12.5 or 25 ng μl −1 , erythromycin at the following concentrations 0.1, 0.5, 1, 5 or 10 (μg ml −1 ), hydrogen peroxide at the following concentrations 0.5 or 5 mM. Cultures were also grown at the following conditions: strict anaerobically (Elektrotek Workstation), room atmosphere or pH at levels 5.5, 6.4, 7.3, 8.1 or 9. Sub-cellular protein isolation Bacteria were generally harvested at exponential (OD 620 nm =0.4–0.5) or at stationary phase (OD 620 nm =0.7–0.8) by centrifugation 10 min at 2,500 g . To isolate intracellular proteins samples were treated as earlier described [1] . For surface-associated protein isolation, TBS washed cells were resuspended in 20 mM Tris–HCl, 150 mM NaCl, 10 mM CaCl 2 , 1 M D -arabinose, pH 7.6 to a concentration of 1.6 × 10 [9] colony forming units per ml. Samples were treated with 10 μg sequencing grade trypsin (Promega) per ml for 15 min at 37 °C (refs 44 , 45 ). Cells were removed by centrifugation at 1,000 g for 15 min at 4 °C and the resulting supernatant was treated as described below in the ‘Protein digestion & peptide cleaning’ section except for more extensive washes during peptide cleaning for arabinose removal. Secreted proteins were isolated from 22 μm filtered culture supernatants that were concentrated with Amicon Ultra-15 Centrifugal Filter Units, 30 MWCO (Millipore). The resulting concentrate was diafiltrated in the same filter unit type twice with 50 mM Tris–HCl, pH 8.35 and then once with 6 M Urea, 0.2 M Tris–HCl, pH 8.35. Protein digestion and peptide cleaning The proteins were reduced with 5 mM dithiothreitol for 45 min at 37 °C, and alkylated with 25 mM iodoacetamide for 45 min before diluting the sample with 100 mM ammonium bicarbonate to a final urea concentration below 1.5 M. Proteins were digested by incubation with trypsin (1/100, w/w) for at least 6 h at 37 °C. The peptides were cleaned up by C18 reversed-phase spin columns according to the manufacturer’s instructions (Harvard Apparatus). Shotgun tandem MS analysis The shotgun tandem and targeted MS analysis was performed as previously described [1] . Briefly, the hybrid Orbitrap-LTQ XL mass spectrometer (Thermo Electron, Bremen, Germany) was coupled online to a split-less Eksigent 2D NanoLC system (Eksigent technologies, Dublin, CA, USA). Peptides were loaded with a constant flow rate of 10 μl min −1 onto a precolumn (Zorbax 300SB-C18 5 × 0.3 mm, 5 μm, Agilent technologies, Wilmington, DE, USA) and subsequently separated on a RP-LC analytical column (Zorbax 300SB-C18 150 mm × 75 μm, 3.5 μm, Agilent technologies) with a flow rate of 350 nl min −1 . The peptides were eluted with a linear gradient from 95% solvent A (0.1% formic acid in water) and 5% solvent B (0.1% formic acid in acetonitrile) to 40% solvent B over 55 min. The mass spectrometer was operated in data-dependent acquisition mode to automatically switch between Orbitrap-MS (from m/z 400 to 2,000) and LTQ-MS/MS. Four MS/MS spectra were acquired in the linear ion trap per each Fourier Transform-MS scan, which was acquired at 60,000 FWHM nominal resolution settings using the lock mass option ( m/z 445.120,025) for internal calibration. The dynamic exclusion list was restricted to 500 entries using a repeat count of two with a repeat duration of 20 s and with a maximum retention period of 120 s. Precursor ion charge state screening was enabled to select for ions with at least two charges and rejecting ions with undetermined charge state. The normalized collision energy was set to 30%, and one microscan was acquired for each spectrum. The data analysis was performed as previously described [1] . Briefly, the resulting MS2 data were searched with X! Tandem search engine, version 2009.04.01.1 with the k -score plugin [46] , a common peptide and protein list was generated using the Trans-Proteomic pipeline, version 4.4.0 (ref. 47 ). All searches were performed with full-tryptic cleavage specificity, up to 2 allowed missed cleavages, a precursor mass error of 15 p.p.m. and an error tolerance of 0.5 Da for the fragment ions. Because of the sample preparation cysteine carbamidomethylation was defined as fixed modification in the search parameters. A protein database with sequences for GAS SF370 (Genome ID 79,812 from PATRIC) was used to match the individual spectra to certain peptides. The database was extended by decoy sequences to validate the resulting peptide-spectrum matches [48] . A 1% false discovery rate (FDR) was then used to generate the final protein list with ProteinProphet. MS1-based quantification was done using SuperHirn [49] . Features were detected using SuperHirn using a RT tolerance of 1, MS1 m/z tolerance of 10, MS2 PPM m/z tolerance of 30. Only features with charge 1–5 were included. Any feature for which >1 peptide could be identified at the 1% FDR, hence mapping to >1 protein, were discarded. Generation of proteome-wide SRM assays We generated experimentally validated SRM assay for three PTPs for each protein in the SF370 proteome. Transitions were generated from experimental MS2 spectra either from Off Gel Electrophoresis fractionated cell lysates for a pool of GAS SF370 grown under various conditions or from crude synthetic peptides purchased from JPT (Berlin, Germany). The transitions were scored in a scoring scheme that favored y-ions over b-ions, required both Q1/Q3 to be between 400 and 1,500 M/Z, Q3 larger than Q1 was favored and precursor charge of two was preferred over other charge states. The four best transitions for each peptide were measured in none-scheduled SRM mode against the sample where the peptide was identified by MS2. SRM analysis SRM transition assays were constructed by testing the twenty most abundant peptide fragments for selected PTPs identified with high confidence in the LC–MS/MS experiments. Spiked in the RT-peptides (Biognosys AG, Zurich, Switzerland) allowed normalization of the RT as previously described [20] . The SRM measurements were performed on a TSQ Vantage triple quadropole mass spectrometer (Thermo Electron, Bremen, Germany) equipped with a nanoelectrospray ion source (Thermo Electron). Chromatographic separations of peptides were performed on an Eksigent 1D NanoLC system (Eksigent technologies) using the same chromatographic conditions as described above for the Eksigent 2D NanoLC system connected to the hybrid Orbitrap-LTQ XL mass spectrometer. The LC was operated with a flow rate of 400 nl min −1 . The mass spectrometer was operated in SRM mode, with both Q1 and Q3 settings at unit resolution (FWHM 0.7 Da). A spray voltage of +1,700 V was used with a heated ion transfer setting of 270 °C for desolvation. Data were acquired using the Xcalibur software (version 2.1.0). The dwell time was set to 10 ms and the scan width to 0.01 m/z . All collision energies were calculated using the formula: CE=(Parent m/z ) × 0.034+3.314. The data analysis was performed as previously described [20] using a 1% FDR. The resulting peptide abundances were exported into a database, where protein abundances were inferred by summing up the abundances for the peptides uniquely mapping to each protein. [22] How to cite this article: Karlsson, C. et al. Proteome-wide selected reaction monitoring assays for the human pathogen Streptococcus pyogenes . Nat. Commun. 3:1301 doi: 10.1038/ncomms2297 (2012).